Microwave purification of large-area horizontally aligned arrays of single-walled carbon nanotubes Recent progress in the field of single-walled carbon nanotubes (SWNTs) significantly enhances the potential for practical use of this remarkable class of material in advanced electronic and sensor devices. One of the most daunting challenges is in creating large-area, perfectly aligned arrays of purely semiconducting SWNTs (s-SWNTs). Here we introduce a simple, scalable, large-area scheme that achieves this goal through microwave irradiation of aligned SWNTs grown on quartz substrates. Microstrip dipole antennas of low work-function metals concentrate the microwaves and selectively couple them into only the metallic SWNTs (m-SWNTs). The result allows for complete removal of all m-SWNTs, as revealed through systematic experimental and computational studies of the process. As one demonstration of the effectiveness, implementing this method on large arrays consisting of ~20,000 SWNTs completely removes all of the m-SWNTs (~7,000) to yield a purity of s-SWNTs that corresponds, quantitatively, to at least to 99.9925% and likely significantly higher. The extraordinary electrical properties [1] , [2] , [3] of semiconducting single-walled carbon nanotubes (s-SWNTs) make them uniquely attractive for use in logic transistors/circuits [4] , [5] , [6] , [7] , [8] , [9] , [10] , radiofrequency (RF) transistors [11] , [12] , [13] , [14] , [15] , [16] , optoelectronic devices [17] , [18] , [19] and sensors [20] , [21] , [22] . The required horizontally aligned array configurations in SWNTs are possible through chemical vapour deposition (CVD)-based growth on quartz substrates [23] , [24] . A long-standing challenge for use of such arrays in demanding applications arises from the need to remove all of the metallic tubes (m-SWNTs), which typically comprise ~1/3 of all of the SWNTs. Techniques for selective growth [25] , [26] and for post-growth purification via chemical etching/separation [27] , [28] , [29] , optical ablation [30] , [31] or electrical breakdown [32] provide some capabilities in yielding s-SWNTs in CVD arrays, but none approaches the daunting requirements in purity for applications in low-power digital circuits (>99.9999% s-SWNTs) [33] . A recently described alternative method referred to as thermocapillary-enabled purification [34] can exceed these targets. Here a partial top-gate transistor structure allows selective current injection into the m-SWNTs. The resulting local Joule heating creates increases in temperature (a few degrees) that lead to gradients (tens of degrees per μm) sufficiently large to drive thermocapillary flow in an overcoat of an amorphous small-molecule material (thermocapillary resist, Tc-resist). This flow forms local trenches above the m-SWNTs, thereby exposing them for complete elimination by reactive ion etching (RIE), without damaging the s-SWNTs. Although effective, this method has several practical disadvantages, such as: the need for multiple deposition and etching steps to form the necessary electrodes and gating structures; the requirement of physical contact with these electrodes to allow selective current injection; and residue and other contamination that often remains, even after removal of these materials following the purification process. To avoid these issues, here we implement a different scheme in which microwave radiation selectively heats the m-SWNTs to levels that initiate the thermocapillary flows. Microwave radiation represents a noninvasive heating technique, which is simple and scalable. For low cost, desktop sources of microwaves, the intensity below the level required for non-negligible direct heating of SWNTs, because of their extremely small absorption cross-sections [35] . Antennas can, however, simultaneously amplify the microwave power and selectively transfer the radiation energy into heating of m-SWNTs. Systematic experimental studies demonstrate the effectiveness of this simple process by complete and selective removal of m-SWNTs from large and small arrays of SWNTs, including examples that include tens of thousands of SWNTs. Measurements and computational results reveal all of the fundamental aspects of interactions between the microwaves, antennas and SWNTs. The results represent substantial progress towards the large-scale, economical production of well-aligned arrays of purely s-SWNTs. Microwave purification of large-area arrays of aligned SWNTs Schematic illustrations and corresponding images for each step of the microwave purification process appear in Fig. 1a,b (i–iii) . Patterning narrow strips of iron catalyst particles on a quartz substrate followed by CVD growth [23] yields nearly perfectly aligned, horizontal arrays of SWNTs that include both metallic and semiconducting types. A second patterning step defines collections of microstrip dipole antennas (typically 50 nm Ti) that amplify the microwave field and effectively transfer incident power into current flows selectively in the m-SWNTs. Without the antennas, the heating of the SWNTs is negligible ( Supplementary Fig. 1 ). Although other antenna geometries can be considered [36] , the designs used here are attractive because of their simple planar layouts. Increasing the lengths of the strips and decreasing their separations improve the field enhancement. The lengths, widths and separations for experiments reported here are L A =500 μm (length of one arm in the dipole), W A =1 mm (width of an arm) and L 0 =15 μm (gap between the arms), respectively. Details appear in Supplementary Fig. 2a . Deposition of a uniform overcoat of Tc-resist (typically ~30 to 40 nm thick) followed by microwave irradiation (300 W, 70 °C, 3 h) in a small, desktop single-mode cavity ( Supplementary Fig. 3 ) initiates mild heating selectively in the m-SWNTs and resulting thermocapillary flows at these locations (increases in microwave power can enable reductions in L A and increases in L 0 , for single-step, rapid purification over areas larger than those described here). The open trenches that form as a result of the flows allow complete removal of the m-SWNTs by RIE, without affecting the s-SWNTs. Washing away the Tc-resist with acetone completes the purification process. 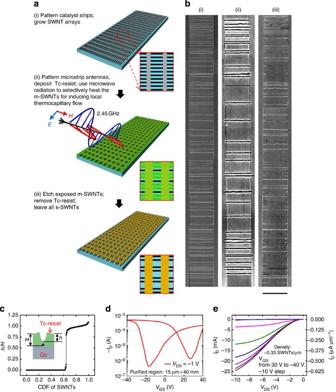Figure 1: Microwave-based purification of large arrays of aligned SWNTs. (a) Schematic illustration of the key steps in the process. (i) CVD growth yields aligned SWNTs of both metallic and semiconducting types. (ii) Microstrip antennas (Ti) defined on this substrate convert incident microwave irradiation into Joule heating selectively in only the m-SWNTs. The resulting heating causes local thermocapillary flow of a thin overcoat (~35 nm) of an amorphous organic material (thermocapillary resist, Tc-resist), thereby opening trenches at the m-SWNTs. (iii) Etching away the exposed m-SWNTs and removing the Tc-resist leaves arrays of pure, unmodified s-SWNTs. (b) AFM and SEM images at each step: (i) pristine arrays of SWNTs before the purification; (ii) topography associated with formation of trenches at the m-SWNTs and (iii) s-SWNTs after the purification. Scale bar, 15 μm. (c) Statistics of the normalized average trench depths (h/H) along each SWNT, plotted as a function of the cumulative distribution fraction (CDF) of the SWNTs (387 in total). The results indicate that ~36% of the SWNTs yield deep trenches. The inset provides a schematic illustration of the geometry for extracting the trench depth, with key parameters defined. (d,e) Cumulative transfer curves and output characteristics for 40 transistors built with purified arrays of SWNTs. The transistors utilize the Ti microstrip antennas as source and drain contacts, with channel lengths ~15 μm and channel widths ~1 mm, to achieve an on/off ratio ~103and large output current ~25 mA. Figure 1: Microwave-based purification of large arrays of aligned SWNTs. ( a ) Schematic illustration of the key steps in the process. (i) CVD growth yields aligned SWNTs of both metallic and semiconducting types. (ii) Microstrip antennas (Ti) defined on this substrate convert incident microwave irradiation into Joule heating selectively in only the m-SWNTs. The resulting heating causes local thermocapillary flow of a thin overcoat (~35 nm) of an amorphous organic material (thermocapillary resist, Tc-resist), thereby opening trenches at the m-SWNTs. (iii) Etching away the exposed m-SWNTs and removing the Tc-resist leaves arrays of pure, unmodified s-SWNTs. ( b ) AFM and SEM images at each step: (i) pristine arrays of SWNTs before the purification; (ii) topography associated with formation of trenches at the m-SWNTs and (iii) s-SWNTs after the purification. Scale bar, 15 μm. ( c ) Statistics of the normalized average trench depths ( h / H ) along each SWNT, plotted as a function of the cumulative distribution fraction (CDF) of the SWNTs (387 in total). The results indicate that ~36% of the SWNTs yield deep trenches. The inset provides a schematic illustration of the geometry for extracting the trench depth, with key parameters defined. ( d , e ) Cumulative transfer curves and output characteristics for 40 transistors built with purified arrays of SWNTs. The transistors utilize the Ti microstrip antennas as source and drain contacts, with channel lengths ~15 μm and channel widths ~1 mm, to achieve an on/off ratio ~10 3 and large output current ~25 mA. Full size image Figure 1c shows the normalized average trench depth ( h/H , where h is the average trench depth and H is thickness of the Tc-resist; see inset schematic in Fig. 1c ) along each SWNT (387 SWNTs investigated across an array with density ~0.5 SWNTs per μm) in the form of a cumulative distribution function (CDF). The results exhibit two distinct regions, that is, no trenches or deep trenches, with a cutoff at CDF~0.64, corresponding to fully developed trenches at ~36% of the SWNTs in the array. This number is close to the expected population (~33%) of m-SWNTs derived from CVD growth. Transistors that utilize the microstrip antennas as source-drain contacts (channel length L ch =~15 μm, channel width W ch =~1 mm; see Supplementary Fig. 2a ) exhibit collective transfer curves and output characteristics ( Fig. 1d,e , from 40 transistors added together; individual transistor responses in Supplementary Fig. 2b ) consistent with complete removal of m-SWNT, that is, ratio of on to off currents of >1,000. High-output currents (~25 mA) are consistent with retention of a large majority of the s-SWNTs. This demonstration involves both large areas (15 μm × 40 mm=0.6 mm 2 ) and numbers of SWNTs (~20,000). The expected current from a single m-SWNT in this device structure (~2–3 μA for V DS =−1 V (refs 37 , 38 ) is much larger than the observed off current (~0.5 μA), thereby suggesting a purity in s-SWNTs of >99.9925% (when one m-SWNT exists among the s-SWNTs, the purity is 1-1/(20,000*2/3)=99.9925%). Effectiveness of microwave purification Criteria for effectiveness of this process include [33] , [39] the elimination of all of the m-SWNTs, and the preservation of all of the s-SWNTs, without change in their intrinsic properties [33] , [39] . To quantify the effectiveness, we exploit detailed imaging (scanning electron microscopy (SEM) and atomic force microscopy (AFM)) and electrical measurements on small arrays of SWNTs (each with between 10 and 31 SWNTs, for easy imaging) before and after the purification (for direct comparisons). The test structures ( Supplementary Fig. 4a,b ) use Ti microstrip antennas ( Supplementary Fig. 5 ) as the source-drain contacts, where poly(methyl methacrylate) (PMMA) serves as the gate dielectric (for easy removal after characterization) and Ti (50 nm) as the gate metal. 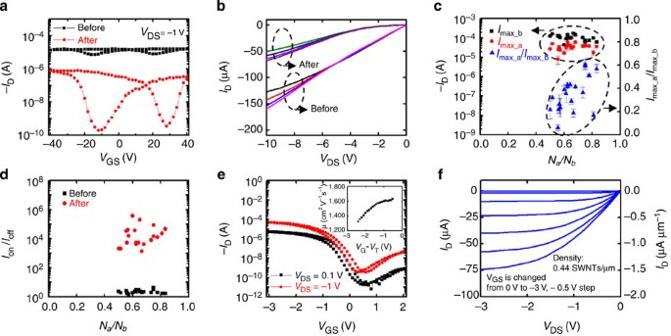Figure 2: The effectiveness of the microwave-based purification process. (a,b) Typical transfer curves and output characteristics (near the on state region) for transistors built on small arrays of SWNTs before and after purification. The transistors use Ti metal as the source and drain electrodes, which also serve as the antennas during the purification. The on/off ratio of the transistors increases from ~2.2 to ~4.2 × 103, and the maximum output current decreases by only ~41%. (c) The maximum output current before and after (Imax_bandImax_a, respectively) purification, as a function of the ratio of the number of SWNTs after purification to the value before purification (Na/Nb).Imax_a/Imax_branges from 0.1 to 0.6, and increases withNa/Nb. The results indicate that the s-SWNTs are well preserved. (d) Statistics of the on/off ratios (Ion/Ioff) of transistors based on the SWNTs before and after the purification, respectively. TheIon/Ioffincreases from <5 to 1 × 103~106, suggesting complete removal of the m-SWNTs. (e,f) Typical transfer curve and output characteristics of a transistor built on a small array of purified SWNTs with Pd contacts and a gate dielectric of SU8 (50 nm)/HfO2(5 nm). The low hysteresis, p-type behaviour facilitates extraction of the device mobility, which is ~1,600 cm2V−1s−1as shown in the inset graph. Figure 2a shows representative transfer characteristics evaluated before and immediately after purification (implemented here in three cycles of Tc-resist deposition and microwave irradiation to improve the yields; details in the Supplementary Note 1 ). In this example, the process removes 8 of 25 SWNTs in the device, thereby increasing the on/off ratio from ~2.2 to ~4.2 × 10 3 . If we assume, as a rough estimate, that the on currents in the s-SWNTs are similar to those of the m-SWNTs at similar bias conditions, then even a single remaining m-SWNT would lead to on/off ratios of <17 (<2.6 if the on currents in the s-SWNTs are ten times smaller than the m-SWNTs [40] , as might be expected because of poor contacts to the s-SWNTs associated with the Ti electrodes). The measured on/off ratio is therefore consistent with complete removal of all m-SWNTs. The relatively large reduction in on current in Fig. 2a (~13.9 to ~0.8 μA) is a consequence of the large Schottky barriers that form at the contacts between the s-SWNT and the Ti [40] , [41] ( Supplementary Fig. 6 ), rather than the degradation of s-SWNTs. Currents measured at high source/drain bias ( I max at V DS =−10 V; Fig. 2b ), where contact effects are minimal ( Supplementary Fig. 7 and Supplementary Table 1 ), indicate a reduction of only ~60%, at various gate voltages ( V GS ). This value is within a range expected for complete retention of the s-SWNTs, with unmodified electrical properties [34] . For 20 transistors studied in this manner, the process removes 143 of 409 SWNTs ( Supplementary Table 2 ). The corresponding percentage (~35%) is consistent with the results of Fig. 1 , and the expected population of m-SWNTs. Moreover, the on-off ratios ( I on / I off ) and the ratios of the numbers of SWNTs before and after purification ( N a / N b ) are consistent with effective operation of the process ( Fig. 2d and Supplementary Table 2 ). The ratio of I max before and after purification ( I max _ b / I max _ a ) ranges from 0.1 to 0.6, and increases with N a / N b ( Fig. 2c ). The large current retention (weighted average value of I max _ a / I max _ b ~0.35) together with the expected, large percentage of remaining SWNTs (65%), provide additional evidence that the process preserves all, or nearly all, of the s-SWNTs. Figure 2: The effectiveness of the microwave-based purification process. ( a , b ) Typical transfer curves and output characteristics (near the on state region) for transistors built on small arrays of SWNTs before and after purification. The transistors use Ti metal as the source and drain electrodes, which also serve as the antennas during the purification. The on/off ratio of the transistors increases from ~2.2 to ~4.2 × 10 3 , and the maximum output current decreases by only ~41%. ( c ) The maximum output current before and after ( I max _ b and I max _ a , respectively) purification, as a function of the ratio of the number of SWNTs after purification to the value before purification ( N a / N b ). I max _ a / I max _ b ranges from 0.1 to 0.6, and increases with N a / N b . The results indicate that the s-SWNTs are well preserved. ( d ) Statistics of the on/off ratios ( I on / I off ) of transistors based on the SWNTs before and after the purification, respectively. The I on / I off increases from <5 to 1 × 10 3 ~10 6 , suggesting complete removal of the m-SWNTs. ( e , f ) Typical transfer curve and output characteristics of a transistor built on a small array of purified SWNTs with Pd contacts and a gate dielectric of SU8 (50 nm)/HfO 2 (5 nm). The low hysteresis, p-type behaviour facilitates extraction of the device mobility, which is ~1,600 cm 2 V −1 s −1 as shown in the inset graph. Full size image Effectively assessing the performance of purified arrays benefits from ohmic contacts (Pd) and high-capacitance gate dielectrics (SU8 (50 nm)/HfO 2 (5 nm)). Transistors with such designs ( Supplementary Fig. 4c ) show p type characteristics with low hysteresis ( Fig. 2e,f ). The results allow quantitative extraction of mobilities. The average values that use rigorous calculations of the gate capacitance [42] , [43] , [44] , [45] ( Supplementary Note 2 ) and neglect contact resistances are ~1,600 cm 2 V −1 s −1 as shown in the inset of Fig. 2e (weighted average ~1,100 cm 2 V −1 s −1 for various devices, Supplementary Fig. 8 ). Mobilities in this range are comparable to those reported from pristine SWNTs 2 on quartz, as well as s-SWNTs purified via TcEP with direct current (DC) injection [34] . Heating mechanisms and origins of selectivity Three-dimensional (3D) finite element analysis (FEA), calculations using an equivalent circuit model and experimental measurements illustrate the mechanisms that underlie the conversion of microwave radiation into selective heating of the m-SWNTs. The first part of the process involves interactions between the microwave fields and the microstrip dipole antennas. 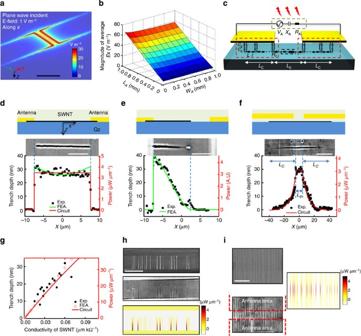Figure 3: Coupling between the microwave field, the antennas and the SWNTs. (a) Finite element analysis (FEA) of the distribution of the electric field around a microstrip dipole antenna, revealing a strong enhancement near the gap between two antenna arms. Scale bar, 65 μm. (b) FEA of the field enhancement as a function of the length and width of the antenna. The enhancement scales approximately linearly with the length of the antenna, whereas it is relatively insensitive to the width. (c) An equivalent circuit for the antenna and SWNT system. (d) Schematic illustration of an individual m-SWNT in contact with both arms of the antenna. The AFM topography image and the plot below show a relatively constant trench depth along the length of the SWNT. The green and red curves correspond to heating profiles from the FEA and circuit models, respectively. Scale bar, 5 μm. (e) Schematic illustration of an individual m-SWNT in contact with only one arm of the antenna. The AFM topography image and trench profile show a decrease in the depth of the trench, starting from the edge of the antenna arm in contact with the SWNT to its opposite end, where the trench gradually vanishes. This trend matches the heating profile predicted by the FEA simulation. Scale bar, 5 μm. (f) Schematic illustration of an m-SWNT under an antenna without direct contact. The AFM topography image and plot of the trench profile are from an m-SWNT in an array of well-separated SWNTs. The trench not only exists in between the two antenna arms, but also extends underneath both arms. The heating profile computed using the circuit model with the resistivity of the SWNT as the only fitting parameter (70 kΩ μm−1) matches the trench profile. Scale bar, 20 μm. (g) Average trench depth along the SWNT, for 16 individual m-SWNT devices, as a function of the resistivity of the SWNT. The open circles and the red curve are heating profiles from the FEA and circuit model, respectively. (h,i) SEM, AFM topography and FEA images of arrays of SWNTs with only one side in contact and without contact, respectively. Scale bars, 15 μm. Figure 3a shows simulated distributions of the magnitude of the electrical field (E-field) near the gap between the antenna arms for normally incident plane waves polarized along the arms (see Supplementary Fig. 9a,b for other polarizations). The results show that large-field enhancements are possible (line plots across the gap appear in Supplementary Fig. 9c ). For the range of dimensions studied here, FEA modelling establishes ( Fig. 3b ) that the enhancement of the average E-field in the X direction ( E X ) increases approximately linearly with L A and decreases slightly with increasing W A and decreasing thickness ( Supplementary Fig. 9d ). The field is inversely proportional to L 0 ( Supplementary Fig. 9c ), consistent with expectation based on simple electrostatics. Figure 3: Coupling between the microwave field, the antennas and the SWNTs. ( a ) Finite element analysis (FEA) of the distribution of the electric field around a microstrip dipole antenna, revealing a strong enhancement near the gap between two antenna arms. Scale bar, 65 μm. ( b ) FEA of the field enhancement as a function of the length and width of the antenna. The enhancement scales approximately linearly with the length of the antenna, whereas it is relatively insensitive to the width. ( c ) An equivalent circuit for the antenna and SWNT system. ( d ) Schematic illustration of an individual m-SWNT in contact with both arms of the antenna. The AFM topography image and the plot below show a relatively constant trench depth along the length of the SWNT. The green and red curves correspond to heating profiles from the FEA and circuit models, respectively. Scale bar, 5 μm. ( e ) Schematic illustration of an individual m-SWNT in contact with only one arm of the antenna. The AFM topography image and trench profile show a decrease in the depth of the trench, starting from the edge of the antenna arm in contact with the SWNT to its opposite end, where the trench gradually vanishes. This trend matches the heating profile predicted by the FEA simulation. Scale bar, 5 μm. ( f ) Schematic illustration of an m-SWNT under an antenna without direct contact. The AFM topography image and plot of the trench profile are from an m-SWNT in an array of well-separated SWNTs. The trench not only exists in between the two antenna arms, but also extends underneath both arms. The heating profile computed using the circuit model with the resistivity of the SWNT as the only fitting parameter (70 kΩ μm −1 ) matches the trench profile. Scale bar, 20 μm. ( g ) Average trench depth along the SWNT, for 16 individual m-SWNT devices, as a function of the resistivity of the SWNT. The open circles and the red curve are heating profiles from the FEA and circuit model, respectively. ( h , i ) SEM, AFM topography and FEA images of arrays of SWNTs with only one side in contact and without contact, respectively. Scale bars, 15 μm. Full size image This E-field initiates movements of free carriers in the SWNTs ( Supplementary Fig. 9e ). The resulting current leads to Joule heating. The wavelength of the microwave radiation (~12.2 cm) is much larger than the dimensions of the system (that is, the antennas, and the SWNTs). As a result, an equivalent circuit model can be implemented under the quasi-static approximation ( Fig. 3c and Supplementary Fig. 10a,b ) to obtain physical insights into the heating mechanisms. Here the electrically small antenna is equivalent to a voltage source ( V A ) with internal resistance ( R A , mainly from resistance of the metal strip) and reactance ( X A , mainly from the capacitance of the antenna), the values of which can be extracted from FEA simulations or analytical calculations ( Supplementary Fig. 10c ). The simplest case corresponds to the presence of a single m-SWNT, treated as a series of lumped resistors ( r , defined as kΩ μm −1 ) and inductors ( L , defined as H m −1 ) [46] . The length of physical overlap between the m-SWNT and the antenna ( L C ) allows electrical coupling through the associated capacitances (geometric and quantum capacitance C g and C q , respectively) and a shunt conductance ( G ). The resulting network of elements has an impedance that can be calculated analytically. By ignoring capacitive coupling between the exposed region ( L 0 ) and the antenna, this segment of the m-SWNT can be treated as a pure load, with impedance of Z 0 =( r + iωL ) L 0 , dominated by the resistance rL 0 . Details of each value are in Supplementary Note 3 . The geometry used for the purification process summarized in Figs 1 and 2 ( Supplementary Fig. 5 ) appears in the schematic illustration near the top of Fig. 3d . The AFM topography image and the graph illustrate the trench morphology and its depth as a function of position along the m-SWNT, respectively. The microwave conditions are 160 W, 70 °C, 3 h and the Tc-resist has a thickness of ~40 nm. Here the trench has a depth that is independent of position along the m-SWNT. The linear relationship between trench depth and heating power ( Supplementary Fig. 11 ) implies a spatially uniform heating profile. Quantitative calculations of the power density from FEA and the circuit model follow from use of the resistance of the m-SWNT ( r =80 kΩ μm −1 ) measured under DC conditions, and simulated microwave radiation (equivalent voltage for the circuit) as the source ( Supplementary Fig. 12 ). The DC value of r provides a good approximation of the corresponding AC value because ωτ ≪ 1, where τ (~10 −12 s) [38] is the characteristic scattering time in SWNTs and ω is the angular frequency of the microwaves (2 π × 2.45 GHz). The simulations show a nearly constant heating profile, consistent with experimental observations of the trench depth. Based on the similarity in flow profiles, the temperature increase associated with microwave irradiation can be assumed to be similar to that associated with DC injection reported previously [34] . Microwave heating power densities between 3 and 30 W m −1 , therefore, correspond to temperature increases at the top-surface of Tc-resist of between 2 and 15 °C (ref. 34 ). In rare cases, the SWNTs make contact only to one side of the antenna, as shown in the Fig. 3e . The corresponding AFM topography image and profile of the trench depth associated with a m-SWNT in this type of configuration (metallic type inferred from the formation of the trench; Tc-resist ~40 nm; microwave conditions: 300 W, 70 °C, 3 h) reveal a spatial decrease in depth, starting from the edge of the antenna arm that contacts the m-SWNT and extending continuously to its tip end. This trend matches the heating profiles calculated by FEA, as shown here in arbitrary units (The profile is nearly invariant with r , for values between 10 and 100 kΩ μm −1 . ). This behaviour indicates that the current flow in the SWNT decreases continuously to zero at the tip, as required by the boundary conditions at that location. Another case of interest, as described subsequently, occurs when the SWNTs span the gap but do not directly contact the antenna, as shown in Fig. 3f . Here only capacitive coupling is important. The AFM topography image and trench depth correspond to a m-SWNT (determined by Raman microscopy) in a sparse array (distances from adjacent SWNTs >3 μm) on a sapphire substrate to facilitate Raman measurements [47] ( Supplementary Note 4 and Supplementary Fig. 13 ). Here microwave exposure (160 W, 70 °C, 3 h) occurs, while antennas ( L A =1,000 μm, W A =80 μm and L 0 =8 μm) on a cover glass are separated by a ~1.1-μm air gap above the SWNTs (see Methods). The results show that the trench depth is largest at the centre region ( L 0 ) and gradually decreases to zero within a distance shorter than the overlap length ( L C ). With r =70 kΩ μm −1 , the circuit model yields a spatial variation in heating power that matches the observed trench depth ( Fig. 3f ). These variations take the form of |sinh 2 ( x / L T )|, where is the transfer length (magnitude ~9.5 μm in this case, Supplementary Note 3 ). As the capacitive coupling mechanism does not require the antennas to contact the SWNTs, it provides an interesting option in purification, as described subsequently. On the other hand, direct contact offers significant benefits in selectivity, also as described subsequently. By comparison to individual SWNTs, implementation with arrays involves additional considerations related to wide variations in the electrical properties of the SWNTs [48] , [49] (chiralities, resistivities) and coupling (electrical, thermal, flow) between them. The circuit model treats each SWNT (the centre part with length L 0 ) as a load with impedance Z 0 , which is dominated by the resistance of the SWNT. Experimental validation of this approach can be accomplished through studies of trenches formed in isolated SWNTs with different resistances. The antennas for these measurements use the structure in Supplementary Fig. 5 with Ti (2 nm)/Pd (48 nm) and L 0 =~8 μm. The experiments involve Tc-resist with thickness of ~50 nm, and microwave conditions of 80 W, 60 °C and 3 h. Figure 3g plots the average trench depth formed with 16 different m-SWNTs as a function of their conductivity evaluated at a bias of 1 V ( Supplementary Fig. 14 ). The linear relationship is consistent with a dominant role of the load impedance, as in the FEA simulation and the equivalent circuit model. Arrays of SWNTs can be viewed as individual SWNTs, electrically connected in parallel. Figure 3h,i shows results obtained with arrays (160 W, 70 °C, 3 h, Tc-resist thickness~40 nm) for the cases of contact on one side and for no contact with the antennas, respectively (contacts on both sides appears in Fig. 1b ). The depths of the trenches are different for each of the SWNTs, likely due to variations in their conductances, per results of Fig. 3g . FEA simulations of the heating power along the lengths of the SWNTs provide some insights. Here the FEA modelling treats the SWNTs as uniform resistors, with overall magnitudes that incorporate the contact effects (quantum contact resistances and Schottky barriers at the contacts) in an ad hoc manner. Quantitative treatments using 1D drift diffusion models, described subsequently, capture the detailed physics of these barriers. The results in Fig. 3h include 7 SWNTs with a small r (53.3 kΩ μm −1 , derived from the total resistance measured on the entire array before isolation from one contact), and 15 SWNTs with large r (5,330 kΩ μm −1 to represent the SWNTs that do not form trenches [17] , [50] ). The magnitudes of the computed power inside each SWNT in the array are directly related to the values of r . For this particular geometry, SWNT–SWNT coupling, although present [44] , does not have a significant effect on the results. The non-contact case ( Fig. 3i ) also shows a distribution of trench depths. Here assignments of SWNTs with various resistivity (50 kΩ μm −1 to represent the most conducting SWNTs [37] ; 150 kΩ μm −1 to represent moderate conducting ones [51] ; 5,000 kΩ μm −1 to represent the least conducting ones [50] ) in the FEA allow correlation of the conductances of the SWNTs with the magnitudes of heating, as also expected from the equivalent circuit results. The purification process relies critically on selective heating in the m-SWNTs. The discussions above relate the resistance of the SWNTs to the heating power imparted into the SWNTs. Although s-SWNTs are generally more resistive than m-SWNTs, unintentional doping [51] , [52] and other effects can diminish these differences. Selectivity in such cases can be greatly enhanced by the Schottky barriers that form at the contacts between the antenna metal and the s-SWNT. These barriers lead to large impedances that block the flow of current (that is, reflect microwave power). Systematic experimental and computational studies of trench formation with antennas constructed using different metals reveal the underlying physics. The investigation begins with a comparison of average currents measured under DC conditions using two terminal test structures (channel length ~15 μm, width ~50 μm, Supplementary Fig. 5 ) formed with various metal contacts, as a means to assess the magnitudes of the Schottky barriers. 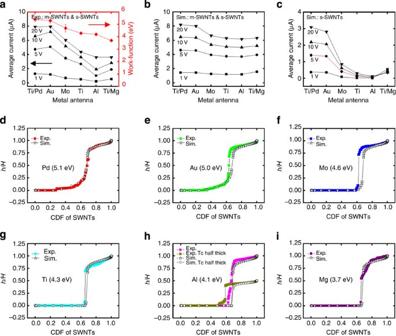Figure 4: Study of the mechanism for selective current injection into the m-SWNTs. (a) Average current per SWNT (black symbols) evaluated in two terminal test structures at bias voltages of 1, 5, 10 and 20 V, for different metals. Data for each metal type correspond to results averaged from more than 100 SWNTs. The average current decreases as the work-function of the metal decreases. (b,c) Simulations of the average current per SWNT for different metal contacts. The simulation averages the currents from SWNTs with different diameters consistent with experimental measurements. Forb, the simulation assumes that one-third of the SWNTs are metallic. Forc, the results involve only s-SWNT. The general trends from simulations match the experimental observations. As the work-function of the contacts decreases, the current in the s-SWNTs decreases due to the formation of the Schottky barriers at the contacts of the s-SWNTs. The slight increase of the current for Mg contact arises from band-to-band tunnelling effects. (d–i) Experimental and simulated statistics of the normalized trench depths for different metals as the antennas during the microwave process, (d) Pd (113 SWNTs), (e) Au (229 SWNTs), (f) Mo (159 SWNTs), (g) Ti (311 SWNTs), (h) Al (337 SWNTs), (i) Mg (170 SWNTs). For metals with relatively high work-function, such as Pd and Au, both the m-SWNTs and some fraction of the s-SWNTs create trenches. For metals with low work-function, such as Mo, Ti, Mg, a distinct onset in the trench depth statistics separate the m-SWNTs from the s-SWNTs. The Al antenna results in a continuous distribution of trench depths, and a gap appears when the thickness of the film decreases to ~20 nm. This result suggests insufficient heating for the m-SWNTs, possibly due to the poor wettability of Al on the SWNTs. The simulations match the experimental results, thereby verifying that the Schottky barrier plays a key role in the selective heating of the m-SWNTs. Figure 4a shows the results, scaled on a per tube basis (each data point averages more than 100 SWNTs) at bias voltages of 1, 5, 10 and 20 V, for different metals (Ti (1 nm)/Pd (49 nm), Au (50 nm), Mo (50 nm), Ti (50 nm), Al (50 nm) and Ti (1 nm)/Mg (70 nm)). The most prominent trend is a decrease in current with work-function, consistent with an increase in the magnitude of the Schottky barriers between the metals and the s-SWNTs. Intrinsic s-SWNTs have a Fermi level at the middle bandgap level ~4.78 eV (ref. 53 ). In practice, s-SWNT often are unintentionally doped (for example, oxygen or water) [17] , [51] , in a way that shifts the Fermi level towards the valence band, to favour hole transport (schematic of band diagram in Supplementary Fig. 15a ). High work-function metal contacts (Pd and Au) are therefore almost transparent to hole injection (schematic band diagram in Supplementary Fig. 15b ). As the work-function decreases, Schottky barriers increase in significance, with an effect of restricting the current flow (schematic band diagram of Mo, Ti, Al, Mg in Supplementary Fig. 15c,d ). Quantitative self-consistent DC drift-diffusion transport simulations support these trends ( Fig. 4b,c , Methods section and Supplementary Note 5 ). The simulations average the currents from SWNTs with different diameters ( Supplementary Fig. 16a ). The results of Fig. 4b assume that one-third of the SWNTs are metallic; Fig. 4c shows results that include only s-SWNTs. As in experiment, decreases in the work-functions increase the Schottky barriers, thereby decreasing the average currents in the s-SWNTs. A slight increase in current for the case of Mg arises from band-to-band tunnelling. The simulations treat the m-SWNTs as the same, in terms of contact properties (the quantum contact resistance h /4 e 2 ), for all metal types. Additional effects such as wettability of the metals on the SWNTs [54] may account for the differences between the measured and simulated current values. To illustrate the significant effects of Schottky barriers on the microwave heating characteristics, squares in Fig. 4d–i show the experimentally measured statistics associated with the normalized trench depths observed in arrays of SWNT with different metal antennas (250 W, 73 °C and 3 h for all metals except Pd, which used 300 W, 70 °C, 3 h; T C -resist thickness~35 nm). The sharp transitions between 0.62 and 0.68 in the CDF for the low work-function metals (Mo, Ti, Al, Mg) are consistent with the experimentally demonstrated selectivity for the case of Ti. The CDF shows smooth variations for high work-function metals (Pd, Au). Al represents an exception to these trends, where sharp and smooth variations occur for Tc-resist thicknesses of ~20 and ~40 nm, respectively. We associate these behaviours with poor wetting of the Al onto the m-SWNT, thereby leading to high contact resistances. Simulation of the heating power (proportional to the trench depth) includes Schottky barriers (derived from the DC transport, see Methods section and Supplementary Note 5 ) in the total impedance calculation (for s-SWNTs). The simulated statistics (stars in Fig. 4d–i , plotted as normalized trench depth) match the observed distribution of trench depths for various metal types investigated here (with the exception of Al, for reasons described above). Detailed studies of the effects of the diameter distributions of s-SWNTs in the grown arrays indicate efficacy in purification across the entire range of diameters when the antennas involve low work-function metals (for details, see Supplementary Fig. 16 ). These experimental and computational studies support the assertion that metals with high work-function (Pd and Au) allow current injection, and therefore Joule heating, in both the m-SWNTs and a portion of the s-SWNTs. Metals with low work-function such as Mo, Ti, Mg, allow current only in the m-SWNTs. The Schottky barriers at the contacts are, therefore, beneficial to selectivity in the purification process. Figure 4: Study of the mechanism for selective current injection into the m-SWNTs. ( a ) Average current per SWNT (black symbols) evaluated in two terminal test structures at bias voltages of 1, 5, 10 and 20 V, for different metals. Data for each metal type correspond to results averaged from more than 100 SWNTs. The average current decreases as the work-function of the metal decreases. ( b , c ) Simulations of the average current per SWNT for different metal contacts. The simulation averages the currents from SWNTs with different diameters consistent with experimental measurements. For b , the simulation assumes that one-third of the SWNTs are metallic. For c , the results involve only s-SWNT. The general trends from simulations match the experimental observations. As the work-function of the contacts decreases, the current in the s-SWNTs decreases due to the formation of the Schottky barriers at the contacts of the s-SWNTs. The slight increase of the current for Mg contact arises from band-to-band tunnelling effects. ( d – i ) Experimental and simulated statistics of the normalized trench depths for different metals as the antennas during the microwave process, ( d ) Pd (113 SWNTs), ( e ) Au (229 SWNTs), ( f ) Mo (159 SWNTs), ( g ) Ti (311 SWNTs), ( h ) Al (337 SWNTs), ( i ) Mg (170 SWNTs). For metals with relatively high work-function, such as Pd and Au, both the m-SWNTs and some fraction of the s-SWNTs create trenches. For metals with low work-function, such as Mo, Ti, Mg, a distinct onset in the trench depth statistics separate the m-SWNTs from the s-SWNTs. The Al antenna results in a continuous distribution of trench depths, and a gap appears when the thickness of the film decreases to ~20 nm. This result suggests insufficient heating for the m-SWNTs, possibly due to the poor wettability of Al on the SWNTs. The simulations match the experimental results, thereby verifying that the Schottky barrier plays a key role in the selective heating of the m-SWNTs. Full size image Purification based on removable antennas Even without the Schottky barriers, however, some level of effectiveness in purification is possible, mainly based on differences between r for m-SWNTs and s-SWNTs ( Supplementary Fig. 17 ). An important opportunity that emerges is the ability to use non-contact, capacitive coupling ( Fig. 3f,i ) with removable and reusable antenna structures ( Supplementary Fig. 18 ). 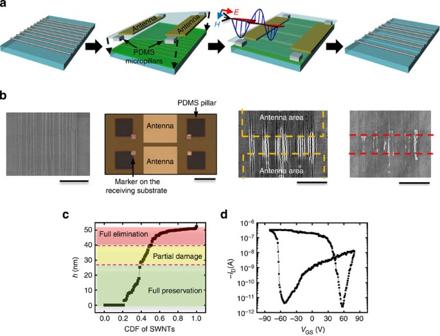Figure 5: Purification based on removable antennas. (a) Schematic illustration of a process that uses removable antennas formed on a glass substrate with PDMS micropillars. Laminating this type of antenna mask on a substrate with aligned SWNTs coated with Tc-resist, followed by microwave irradiation results in sufficient heating to create deep trenches at the m-SWNTs. The micropillars hold the antenna mask and substrate together at a constant distance during the process. The mask can be removed afterward, for reuse. (b) Images corresponding to each step shown in the schematic illustrations: SEM image of the SWNTs before the purification (scale bar, 15 μm); optical image of the antenna mask after contacting the quartz substrate (scale bar, 50 μm); AFM topography image of the trench formation and SEM image after the etching and washing away the Tc-resist (scale bars, 15 μm). (c) Cumulative distribution function of the average trench depths (averaged onL0=8 μm) for 112 SWNTs. The continuous distribution of trench depths suggests that both m-SWNTs and some fraction of the s-SWNTs generate heat to create trenches. As a result, all m-SWNTs and a portion of s-SWNTs can be removed, depending on the trench depths, which are marked in regions that correspond to full elimination (judged by AFM and SEM), partial elimination (judged by SEM and empirical evidence from electrical probing) and full preservation. (d) Transfer curve from a typical transistor that uses arrays of SWNTs purified with an antenna mask. Figure 5a shows a schematic illustration of such a process. Microstrip dipole antennas patterned on a glass substrate with micropillars of poly(dimethylsiloxane) (PDMS) form an ‘antenna mask’. This mask can be laminated on a substrate that supports an array of SWNTs with an overcoat of Tc-resist. Exposure to microwave radiation leads to heating at sufficient levels to create deep trenches at the m-SWNTs for their removal by RIE. The micropillars hold the antenna mask and substrate together at a constant separation distance (set by the height of the micropillars) during the exposure. The mask can be peeled away for re-use ( Supplementary Fig. 19 ). Figure 5b shows a corresponding series of images, including an SEM of the SWNTs before purification; an optical image of the antenna mask in contact with the SWNT substrate (quartz); AFM topography image of the trenches and the SWNTs after etching. The separation between the antennas ( L A =1,500 μm, W A =80 μm, Ti (2 nm)/Pd (48 nm)) and the quartz substrate is ~1.1 μm during the exposure (Tc-resist ~50 nm; microwave conditions: 80 W, 60 °C, 3 h). The CDF of the trench depths (averaged on the centre segment L 0 =8 μm) for 112 SWNTs appears in Fig. 5c . The smooth distribution is consistent with the absence of Schottky barriers that would result from physical contact. In this case, the heating characteristics depend mainly on the values of r and the capacitive coupling strength between the antenna and the SWNTs, as estimated from the equivalent circuit model ( Supplementary Fig. 17 ). As a result, trenches form at some portion of the s-SWNTs. In a practical sense, all m-SWNTs and some of the s-SWNTs can be removed completely; different regions of operation correspond to complete removal (judged by AFM and SEM), partial removal (judged by SEM and empirical evidences from electrical probing) and complete preservation, as illustrated in Fig. 5c . Measurements on transistors built using small arrays of SWNTs (channel length=30 μm, width=35 μm, source-drain contacts Ti (2 nm)/Pd (48 nm), dielectric SU8 2002=2 μm) purified in this manner verify these behaviours ( Fig. 5d ). The extent of removal of s-SWNT can be minimized by eliminating any unintentional doping [55] , a capability that is likely important, in any case, for practical use of s-SWNTs in electronic circuits. The removable antenna is advantageous, because it eliminates the need to perform any processing on the SWNT substrate. Further improvements in its selectivity will make this approach the technique of choice for microwave purification. Figure 5: Purification based on removable antennas. ( a ) Schematic illustration of a process that uses removable antennas formed on a glass substrate with PDMS micropillars. Laminating this type of antenna mask on a substrate with aligned SWNTs coated with Tc-resist, followed by microwave irradiation results in sufficient heating to create deep trenches at the m-SWNTs. The micropillars hold the antenna mask and substrate together at a constant distance during the process. The mask can be removed afterward, for reuse. ( b ) Images corresponding to each step shown in the schematic illustrations: SEM image of the SWNTs before the purification (scale bar, 15 μm); optical image of the antenna mask after contacting the quartz substrate (scale bar, 50 μm); AFM topography image of the trench formation and SEM image after the etching and washing away the Tc-resist (scale bars, 15 μm). ( c ) Cumulative distribution function of the average trench depths (averaged on L 0 =8 μm) for 112 SWNTs. The continuous distribution of trench depths suggests that both m-SWNTs and some fraction of the s-SWNTs generate heat to create trenches. As a result, all m-SWNTs and a portion of s-SWNTs can be removed, depending on the trench depths, which are marked in regions that correspond to full elimination (judged by AFM and SEM), partial elimination (judged by SEM and empirical evidence from electrical probing) and full preservation. ( d ) Transfer curve from a typical transistor that uses arrays of SWNTs purified with an antenna mask. Full size image The schemes presented here provide straightforward, scalable and effective routes to aligned arrays of purely s-SWNTs, with minimal processing. The significant reduction and, for removable antenna approaches, the complete elimination of processing on the nanotube substrate for microwave purification represent significant simplifications compared with previously described Joule heating approaches [34] using electrode structures for gate modulation. The method here is uniquely well suited for use with aligned arrays of SWNTs on solid substrates, where the nanotubes are optimally configured for direct integration into devices with conventional designs. Although not directly applicable to bulk SWNTs, the levels of purity in s-SWNTs that can be achieved significantly exceed those currently possible with other techniques, and there is no need for any solution separation or chemical modification of the SWNTs [56] . All aspects of the purification process are scalable to large areas, and we did not observe any residues associated with etching the m-SWNT (Residue can sometimes arise from photoresist processing and removal of the Tc-resist.). The resulting arrays are well configured for use in various applications, ranging from sensors to low noise RF amplifiers. With sufficiently powerful microwave sources, it may be possible to eliminate the antenna structures entirely ( Supplementary Fig. 1 ), thereby further simplifying the process. Under optimized conditions trench widths of 100–200 nm (ref. 34 ) should be possible ( Supplementary Fig. 20 ), thereby enabling arrays with densities up to ~5 SWNTs per μm. Significantly improved densities should be possible with arrays that have enriched content of semiconducting SWNTs realized by selective growth techniques [25] , [26] . Growing horizontally aligned SWNTs The growth process began with preparation of substrates by cutting quartz wafers (ST-cut; Hoffman) into dies (1.65 cm × 6.5 cm; Disco DAT-6TM dicing saw), and annealing them for 16 h at 900 °C in air. Photolithographic patterning of resist (AZ 5214 positive photoresist), deposition of metal (Fe, 0.2~0.8 nm; electron-beam evaporation, AJA) and lift-off processing defined strips of catalyst (10 μm wide, spaced by 200 μm) oriented perpendicular to the preferred growth direction on the quartz. Annealing the substrate at 950 °C in air for 1 h, cooling to room temperature and then heating to 925 °C again under a flow of H 2 (200 s.c.c.m.) prepared the catalysts for growth. Finally, introducing ethanol (bubbled from a flask at 0 °C by 30 s.c.c.m. H 2 and 30 s.c.c.m. Ar) into the growth tube at 925 °C for 30 min yielded horizontally aligned arrays of SWNTs. Purification via microwave induced thermocapillary flows Photolithography (AZ 2020 negative photoresist), electron-beam evaporation (Ti 50 nm, AJA) and lift-off defined arrays of microstrip antennas. RIE (100 mTorr, 19.6 s.c.c.m. O 2 , 100 W, 45 s; Plasma-Therm RIE) through a photoresist mask (AZ 5214) removed SWNTs everywhere except for regions between the gaps of the microstrip antennas. Thermal evaporation (Kurt Lesker) yielded a uniform, thin layer (typically 30–50 nm) of Tc-resist α,α,α'-Tris(4-hydroxyphenyl)-1-ethyl-4-isopropylbenzene (TCI International). Placing the coated substrate into a 10-ml vial purged with inert gas (Ar) provided a consistent environment for microwave exposure. Transferring the vial to the microwave oven (CEM discovery SP) enabled exposure under controlled conditions (power, maximum temperature and time; a summary of microwave exposure conditions for all experiments described in the main text appears in Supplementary Fig. 21 ). An infrared sensor monitored the temperature of the vial during the experiments. Cooling the vial with a constant flow of nitrogen during exposure helped to maintain a constant temperature. A set of schematic illustrations and optical images of the reactor and the position of the sample and the temperature sensor appear in Supplementary Fig. 3 . After microwave radiation and associated thermocapillary flow, RIE (10 mTorr, 1 s.c.c.m. O 2 , 1 s.c.c.m. CF 4 , 60~80 W, 17 s; Plasma-Therm RIE) removed the exposed m-SWNTs, without affecting the s-SWNTs. Stripping away the Tc-resist with acetone completed the process of forming arrays of purely s-SWNTs. Fabrication and measurement of transistors Fabrication of large-scale transistors (channel length L ch =15 μm, channel width W ch =1 mm) based on large-area, purified arrays of SWNTs used Ti microstrip antennas as the source-drain electrodes. Spin-coating PMMA (950 A7, 1,500 r.p.m. for 45 s and then 4,000 r.p.m. for 30 s, baking 10 min at 110 °C) as the dielectric, and depositing Ti (50 nm) as the top-gate through a shadow mask completed the fabrication processes. Forming transistors ( L ch =15 μm, W ch =50 μm) with pristine, small arrays of SWNTs followed the same procedures described above. After measurements (semiconductor parameter analyzer; Agilent, 4155C), immersing the transistors into acetone removed the PMMA and lifted-off the top-gates. Microwave and etching processes eliminated the m-SWNTs from the arrays. After purification, transistors fabricated with the s-SWNTs facilitated direct comparisons of electrical properties with those from the as-grown, unpurified SWNTs. To obtain transistors with low hysteresis and low operating voltages, photolithography (AZ 2020 negative photoresist) and electron-beam evaporation (2 nm Ti, 48 nm Pd) defined fresh contacts ( L ch =5 μm, W ch =65 μm) on the purified arrays. Spin-casting a thin layer of an epoxy photoresist (diluted SU8, SU8 2000.5: cyclopentanone=1:7; 3,000 r.p.m. for 30 s~50 nm), then baking at 175 °C for 1 h in glove box formed the first layer of the dielectric. Atomic layer deposition (120 °C; Cambridge NanoTech) of HfO2 (5 nm) formed the second layer. Finally, lithography (AZ 5214), electron-beam evaporation (50 nm Ti) and lift-off defined the gate electrode. Forming two-terminal (2T) devices with individual SWNTs derived from arrays of SWNTs with low density (0.1–0.3 SWNTs per μm) followed similar procedures. After forming the contacts, photolithography (AZ 5214) and subsequent RIE (100 mTorr, 19.6 s.c.c.m. O 2 , 100 W, 45 s) removed all of the SWNTs except those protected by narrow regions (~3 μm in width). Scanning electron microscopy (SEM, Hitachi, S-4800) and electrical analyses (Agilent, 4155C) further defined a subset of devices with only a single SWNT bridging the electrodes. Fabricating and characterizing transistors based on such 2T devices used gates on PMMA gate dielectrics, as described previously, to identify the m-SWNTs and s-SWNTs from the electrical responses. Fabricating and applying removable antenna masks Removable antenna masks used cover glass (gold seal, No.1, 0.13–0.17 mm thick; Fisher Scientific) as the supporting substrates, and molded micropillars of PDMS as the adhesive media. The fabrication began with patterning the metal antennas (Ti 50 nm or Ti 2 nm/Pd 48 nm), and then depositing a thin overcoat of SiO 2 (40 nm). Subsequent photolithography defined square windows on another cover glass to form the mold. Spin-casting (4,000 r.p.m., 60 s) a layer of diluted PDMS (two components mixed with 1:30 weight ratio, then diluted by Hexane with 1:16 volume ratio) onto the base, and then attaching the mold to the base in a mask aligner (MJB 4, Suss Microtec) enabled the molding process. The base and mold were transferred into a vacuum chamber (1 × 10 −4 Torr, 10 min) to release trapped air bubbles. Baking on a hot plate (120 °C, 8 h) fully cured the PDMS. Immersion in acetone for overnight dissolved the photoresist on the mold. Peeling off the base and cutting it into dimensions to match the quartz substrates formed the antenna mask. Application of a mask to a substrate with arrays of SWNTs (patterned into lengths of 80 μm) and Tc-resist relied on aligned transfer-printing. The PDMS micropillars held the mask and the sample together with a constant distance (determined by the height of the micropillars and the thin PDMS layer underneath, Supplementary Fig. 18 ) during microwave exposure. After exposure, the antenna mask was simply removed. Modelling of thermocapillary flow The physics of thermocapillary flow can be described by the one-dimensional lubrication equation, where h ( x , t ) is the film thickness, γ is the surface tension, which usually depends linearly on the surface temperature T of film (that is, γ = γ 0 − γ 1 ( T −273)) where γ 0 is the surface tension at 273 K and γ 1 is the temperature coefficient of surface tension, τ =(∂ γ )/(∂ T )(∂ T )/(∂ x ) is the thermocapillary stress, and η is the film viscosity. The initial condition is h ( x , t =0)= h 0 , where h 0 is the initial film thickness, and the boundary conditions are h ( x =±∞, t )= h 0 and ∂ 2 h /∂ x 2 ( x =±∞, t )=0 (zero pressure). The power absorbed by the SWNTs is the summation of a steady-state component Q 0 (power per unit length) and a time-oscillating component Q ( t ) with the frequency on the order of GHz. The thermal diffusion length is defined by , where α is the thermal diffusivity of the film and f is the frequency of microwave radiation. α is usually on the order of 10 −7 m 2 s −1 for a polymer. For f on the order of 1 GHz, the thermal diffusion length is less than 1 nm, which is much smaller than the film thickness (~30 nm) such that the time-oscillating component of power yields a negligible surface temperature rise. Therefore, the surface temperature in equation (1) is mainly from the steady-state power Q 0 and is given by [34] where T 0 is the background heating, L is the SWNT length, k s and k f are the thermal conductivity of substrate and film, respectively, and J 0 is the 0th order Bessel function of the first kind. Here k f =0.2 W m −1 K −1 and k s =6 W m −1 K −1 (refs 34 , 57 ). As the Tc-resist used in the experiment exhibits similar behaviour as polystyrene with a molecular weight 1,215 g mol −1 , we take polystyrene’s surface tension with γ 0 and γ 1 as 47.4 × 10 −3 N m −1 and 0.078 × 10 −3 N m −1 K −1 (ref. 58 ), and viscosity , where T has the unit of K, in our calculations. The Fortran solver PDE_1D_MG can be used to solve equation (1) to yield the evolution of the film thickness h ( x , t ). FEA of the microwave field distributions Three-dimensional finite element simulations (COMSOL, RF module) yielded distributions of the microwave field around the antennas. Implementation of the scattering field formalism with plane waves (normalized E-field 1 V m −1 , polarized along the length of the dipole antenna) as the background field served as the platform for calculations of individual antennas. Treating the microstrip antenna and the SWNT with transition boundaries (thickness 50 nm) simplified the meshing while retaining the essential physics. Because of practical constraints in meshing, the SWNTs were modelled as 50 or 200 nm wide strips (with resistivity scaled to match the resistance of the SWNTs per unit length). Perfectly matched layers enclosing the simulation domain ensured no reflections of the scattered waves. Calculations of antenna arrays utilized the perfect electrical conductor and perfect magnetic conductor conditions for the boundaries perpendicular to the background E-field and M-field, respectively, to guarantee periodicity. Scattering boundary conditions imposed at the upper and lower boundaries absorbed the scattered waves. The calculated E-field (within the middle gap L 0 ) of the antenna arrays differed by ~2% from that of individual antenna for the typical structure ( L A =500 μm, W A =65 μm, L 0 =15 μm, spacing between antennas in the array=1,200 μm). DC transport simulation for different metals as contacts The average current and total resistances of the SWNTs are determined by solving self-consistently the 3D electrostatics and the 1D drift-diffusion transport through the SWNTs. The 3D electrostatics accounts of the full device geometry: the SWNTs on the quartz substrate are terminated by source (S) and drain (D) contacts, and covered by insulating material Tc-resist. The results show that carrier transport depends sensitively on (i) the diameter of the tubes within the as-growth array, (ii) the work-function of the contact materials (Pd (5.1 eV), Au (5.0 eV), Mo (4.6 eV), Ti (4.33 eV), Al (4.1 eV), and Mg (3.7 eV)) [40] , [54] , [59] and (iii) effective applied bias, V DS (extracted by correlating the equivalent trench depths in Tc-resist for DC and microwave inputs). The source to drain of this two-terminal device is separated by L 0 =15 μm. These S/D contacts to the s-SWNTs may involve Schottky barriers (work function of the contact<(electron affinity+band gap) of the s-SWNT) or they can be ohmic (work function of the contact>(electron affinity+band gap) of the s-SWNT). For the s-SWNTs, irrespective of the contact type, we solve the electrostatics and charge density self-consistently [17] , [50] . We find that for the ohmic contact, the electrostatic potential drops linearly through the channel, as expected; whereas, for the Schottky contact, the potential drop depends on the contact resistance and a self-consistent solution between electrostatic potential and charge density is essential. For low Schottky barriers (related to high work function contacts), the current is primarily thermionic; for very high Schottky barriers (related to low work function contacts), the band-bending close to the source contact can be significant enough to induce additional band-to-band tunnelling current [50] . We note that the model is predictive because each component of the model has been validated against independent experiments [17] , [50] . A detailed description of the model follows. Carrier transport in s-SWNT . The electrostatics potential, V , is a solution of Poisson equation, Here the dielectric constant of the medium is ε . The charge density, ρ , is a function of the density of carriers (electron and hole), and fixed interface charges (4.4 × 10 19 cm −3 ) [17] . The fixed charges are determined by fitting the I – V characteristics for one SWNT and subsequently kept constant for all other simulations involving different diameters and contact work function. The electron and hole concentrations must be calculated as a solution of the continuity and the drift-diffusion equations, as follows. Where R is the direct band-to-band recombination rate, q is the electron charge, X is the position variable along the SWNTs, and G SBT,n(p) and G BTBT,n(p) are the generation rate in the channel for electron (hole) because of Schottky-barrier tunnelling and band-to-band tunnelling, respectively, from the source and drain contacts. The expressions for G SBT,n(p) and G BTBT,n(p) along the s-SWNT are Here A =1.5 × 10 2 E G A cm −2 K −2 is the Richardson constant, k B is the Boltzmann constant, T is the lattice temperature and r is a position variable along the SWNTs. Effective mass of electron and hole is m = E G m 0 /20, where m 0 is the mass of free carrier. η n,S(D) =( E F,S(D) − E C )/ k B T , η p,S(D) =( E V − E F,S(D) )/ k B T , E rX ,C = E C ( r )− E C ( X ), E rX ,V = E V ( X )− E V ( r ), where E F,S(D) is the Fermi energy for carriers in S(D) contact. From equation (6) ħ is the reduced Planck’s constant, t is the wall thickness of the SWNT, |d V /d X | is the local electric field along SWNT. The Fermi velocity ( v F =10 8 cm s −1 ) depends the band structure of the SWNTs [17] . The band gap of s-SWNTs is related to the diameter of the tubes ( d ) as E G =0.7/ d eV and δ is the ideality factor. The drift-diffusion currents for electron (hole), I n(p) in equation (4) is represented as, Here I D = I n + I p is the current through the s-SWNT. The field-dependent mobility is μ FE = μ peak /(1+ μ peak |( dV / dX )|/ v s ), where the peak mobility, μ peak =1,600(300/ T )( d /1 nm ) [2] , and v s is the carrier’s saturation velocity [60] . D n(p) is the electron (hole) diffusion coefficient. Additional information including boundary conditions for Poisson and charge continuity and simulation procedures is provided in Supplementary Note 5 . Carrier transport in m-SWNT . Regardless the S/D work function, metallic carbon nanotubes form ohmic contact with source and drain. The electrostatic potential drops linearly within the channel and charge carriers drift in this potential profile. The current through the m-SWNT can be calculated as I D =(4 q 2 / h )( λ eff / L 0 ) V DS (ref. 38 ), where λ eff is the effective mean free path and h is the Planck’s constant. The parameter λ eff can be expressed through Mathiessen’s rule as λ eff −1 = λ e −1 + λ T −1 , where λ e is the elastic scattering mean free path and λ T is the distance an electron must travel in the electric field to reach threshold scattering energy ( ħ Ω) to emit an optical phonon ( ħ Ω=0.2 eV) or zone boundary phonon ( ħ Ω=0.16 eV) [38] . Specifically, λ T = ħ Ω/ qE X , where E X =V DS /L 0 is the average electric field along the m-SWNT. The current flow through the m-SWNT, therefore, is I D =(4 q 2 / h )( λ e E X /(1+ qλ e E X / ħ Ω)). The elastic scattering mean free path is proportional to the m-SWNT diameter through the relation λ e =300 d (ref. 37 ). Once we know the current through each s-SWNT and m-SWNT (discussed above), we calculate the average current for as-grown array SWNTs using the diameter distribution obtained from experiments ( Supplementary Fig. 7a of ref. 17 ). The average current for the as-grown array is computed as ∑ i [ I D( i ) s−SWNT * PDF i *0.67+ I D( i ) m−SWNT * PDF i *0.33]/∑ i [ PDF i *0.67+ PDF i *0.33], where, i is the SWNT index. The average current of an array composed exclusively of s-SWNT is ∑ i I D( i ) s−SWNT * PDF i /∑ i PDF i . We compute the total power dissipation due to joule heating by integrating of the product of the current and local-field along the SWNT, and assume that the heating and the trench-depth are linearly correlated to the power dissipation along the channel. Finally, to differentiate between s-SWNTs versus m-SWNTs, we obtain the CDF of diameter distribution of the as-grown array SWNTs by integrating the probability density function ( Supplementary Fig. 7a of ref. 17 ) and normalizing it to 1. We subdivide CDF in a 2:1 ratio and assign the corresponding fractions to s-SWNTs (0–67%) and m-SWNTs (68–100%). How to cite this article : Xie, X. et al. Microwave purification of large-area horizontally aligned arrays of single-walled carbon nanotubes. Nat. Commun. 5:5332 doi: 10.1038/ncomms6332 (2014).